A novel pathway for the production of hydrogen sulfide fromD-cysteine in mammalian cells In eukaryotes, hydrogen sulphide acts as a signalling molecule and cytoprotectant. Hydrogen sulphide is known to be produced from L- cysteine by cystathionine β-synthase, cystathionine γ-lyase and 3-mercaptopyruvate sulfurtransferase coupled with cysteine aminotransferase. Here we report an additional biosynthetic pathway for the production of hydrogen sulphide from D- cysteine involving 3-mercaptopyruvate sulfurtransferase and D -amino acid oxidase. Unlike the L- cysteine pathway, this D -cysteine-dependent pathway operates predominantly in the cerebellum and the kidney. Our study reveals that administration of D -cysteine protects primary cultures of cerebellar neurons from oxidative stress induced by hydrogen peroxide and attenuates ischaemia-reperfusion injury in the kidney more than L- cysteine. This study presents a novel pathway of hydrogen sulphide production and provides a new therapeutic approach to deliver hydrogen sulphide to specific tissues. Hydrogen sulphide (H 2 S) modulates synaptic activity by enhancing the activity of N -methyl- D -aspartate receptors in neurons and by activating astrocytes that surround the synapse [1] , [2] . It relaxes vascular smooth muscle by activating K + channels and regulates the release of insulin [3] , [4] , [5] , [6] , [7] . In addition to its function as a signalling molecule, H 2 S has a cytoprotective effect. It protects neurons from oxidative stress by recovering glutathione levels, scavenging ROS and suppressing intracellular Ca 2+ concentrations [8] , [9] . This finding led to the identification of H 2 S-mediated cardio- and renal-protection from ischaemia-reperfusion injury [10] , [11] . Most studies about the production of H 2 S have been concentrated on two pyridoxal 5′-phospate-dependent enzymes, cystathionine β-synthase (CBS) and cystathionine γ-lyase (CSE) [1] , [3] , [12] , [13] . Recently, 3-mercaptopyruvate sulfurtransferase (3MST)/cysteine aminotransferase (CAT) pathway has emerged as the third pathway. 3MST produces H 2 S from 3-mercaptopyruvate (3MP), which is generated by CAT from L- cysteine and α-ketoglutarate (α-KG) in the presence of the cofactors thioredoxin and dihydrolipoic acid [14] , [15] , [16] . D- Amino acid oxidase (DAO) can also produce achiral α-keto acids, including 3MP, from D- amino acids, some of which are found in mammalian tissues [17] , [18] , [19] . DAO is localized to peroxisomes, whereas 3MST is mainly found in mitochondria [14] , [20] . Mitochondria and peroxisomes, which are essential cellular organelles in mammals, exchange various metabolites as well as enzymes via a specific form of vesicular trafficking, and are usually in close proximity to each other or have physical contact [21] . 3MST along with DAO can produce H 2 S by the interaction of both organelles. The present study identifies a novel pathway for H 2 S production from D -cysteine and its cytoprotective role in the cerebellum and the kidney. H 2 S production from D -cysteine When we examined the production of H 2 S from brain homogenates, we found that H 2 S was produced from D- cysteine, a negative control for L- cysteine ( Fig. 1a ). Although H 2 S is produced from D- cysteine in microorganisms and plants [22] , its production in mammals is not well understood. Therefore, we compared the catabolism of D- cysteine with that of L- cysteine. The production of H 2 S from D -cysteine was optimal at pH 7.4, whereas production from L -cysteine was greatest at pH 8.4 ( Fig. 1b ). Next, we examined the PLP-dependent nature of the reaction because H 2 S production from L- cysteine by 3MST/CAT and CBS depends on PLP [1] , [14] , [15] . Our results revealed that hydroxylamine, which is an inhibitor of PLP-dependent enzymes, did not have an effect on H 2 S production from D -cysteine except for at 0.5 mM ( Fig. 1c ). At 0.5 mM the production of H 2 S from D -cysteine was increased probably due to the decrease in the competition for D -cysteine with PLP-dependent enzymes, which were greatly suppressed at 0.5 mM. However, at 5 mM, pH of the medium was shifted to acidic, which suppressed H 2 S production from D -cysteine. A single freeze-thaw cycle differently affected enzymatic activity of the two pathways. Specifically, the H 2 S production from D- cysteine was greatly increased, whereas L- cysteine catabolism was decreased ( Fig. 1d ). These observations suggest that the H 2 S-producing pathway from D- cysteine is independent of PLP and distinct from the pathways involving L- cysteine. 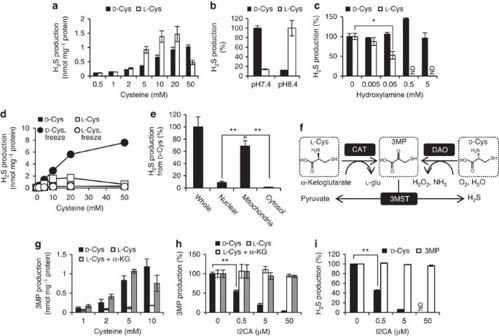Figure 1 H2S-producing activity in the brain usingD-cysteine andL-cysteine as substrates. (a) Production of H2S fromD-cysteine andL-cysteine in brain homogenate. (b) The optimal pH for H2S-producing activities. Potassium phosphate buffer was used for pH 7.4, and Tris/HCl buffer for 8.4. (c) PLP dependency of H2S-producing activity. *P<0.05. (d) The stability of H2S-producing activities following a freeze-thaw cycle. Homogenates that were prepared from brains treated with or without a single freeze-thaw cycle were incubated withD-cysteine orL-cysteine. (e) Localization of H2S-producing activities in the brain. Each fraction was incubated with 10 mMD-cysteine. The whole-brain activity (0.67 nmol mg−1protein) was taken as 100%. **P<0.01. (f) Schematic representation of H2S-producing pathways. (g) The 3MP-producing activities of the homogenates of mitochondrial fraction. Endogenous 3MP contents were subtracted. 3MP (h) and H2S (i) production fromD-cysteine was suppressed by indole-2-carboxylic acid (I2CA). The mitochondrial homogenates were incubated with 10 mMD-cysteine orL-cysteine or 2.5 mM α-ketoglutarate (α-KG). *P<0.05; **P<0.01. All data are represented as the mean±s.e.m. of at least three experiments. Figure 1 H 2 S-producing activity in the brain using D- cysteine and L- cysteine as substrates. ( a ) Production of H 2 S from D- cysteine and L- cysteine in brain homogenate. ( b ) The optimal pH for H 2 S-producing activities. Potassium phosphate buffer was used for pH 7.4, and Tris/HCl buffer for 8.4. ( c ) PLP dependency of H 2 S-producing activity. * P <0.05. ( d ) The stability of H 2 S-producing activities following a freeze-thaw cycle. Homogenates that were prepared from brains treated with or without a single freeze-thaw cycle were incubated with D- cysteine or L- cysteine. ( e ) Localization of H 2 S-producing activities in the brain. Each fraction was incubated with 10 mM D- cysteine. The whole-brain activity (0.67 nmol mg −1 protein) was taken as 100%. ** P <0.01. ( f ) Schematic representation of H 2 S-producing pathways. ( g ) The 3MP-producing activities of the homogenates of mitochondrial fraction. Endogenous 3MP contents were subtracted. 3MP ( h ) and H 2 S ( i ) production from D- cysteine was suppressed by indole-2-carboxylic acid (I2CA). The mitochondrial homogenates were incubated with 10 mM D- cysteine or L- cysteine or 2.5 mM α-ketoglutarate (α-KG). * P <0.05; ** P <0.01. All data are represented as the mean±s.e.m. of at least three experiments. Full size image The DAO-3MST pathway produces H 2 S from D- cysteine We subsequently determined the subcellular localization of the activity to identify the specific pathway involved in the production of H 2 S from D- cysteine. We concluded that ~70% of the H 2 S-producing activity was localized to the mitochondrial fraction, which includes peroxisomes as well as mitochondria ( Fig. 1e ). As mitochondrial 3MST produces H 2 S from 3MP, the existence of an enzyme that produces 3MP from D- cysteine was predicted. It has been previously proposed in hepatocytes that DAO produces 3MP ( Fig. 1f ) [19] . Indeed, 3MP was produced from D- cysteine in the presence of the mitochondrial fraction, and the production was suppressed by the DAO inhibitor indole-2-carboxylate (I2CA) ( Fig. 1g ) [23] . Although 3MP was also produced from L -cysteine with α-KG or L -cysteine alone to a lesser extent, the production was not suppressed by I2CA. In addition, H 2 S production from D- cysteine was suppressed by I2CA, whereas that from 3MP was not ( Fig. 1i ). These observations suggest that DAO uses D- cysteine to produce 3MP, which is in turn metabolized to H 2 S by 3MST. We next utilized recombinant 3MST and DAO to confirm the production of H 2 S via the 3MST/DAO pathway. The results with the recombinant proteins mimicked the endogenous results obtained with the mitochondrial fraction ( Supplementary Fig. S1 ), confirming that the 3MST/DAO pathway produces H 2 S from D- cysteine. Tissue localization of DAO and 3MST Subsequently, the tissue localization of DAO and 3MST was examined by western blot analysis. DAO mostly localized to the cerebellum and the kidney, and 3MST was also found in both tissues ( Fig. 2a–d ). We next examined whether the production of H 2 S from D- cysteine correlated with the localization of DAO and 3MST. Indeed, H 2 S was mainly produced from D- cysteine in the cerebellum and kidney homogenates ( Fig. 2e ). These observations suggest that H 2 S is mainly produced by the 3MST/DAO pathway from D- cysteine in the cerebellum and the kidney. 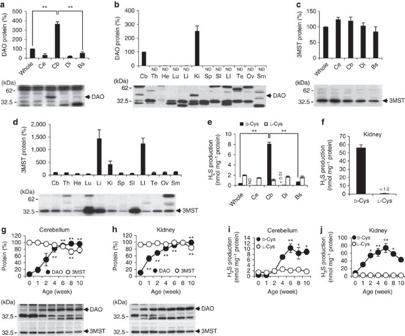Figure 2 Tissue localization of DAO and 3MST and developmental changes in H2S production. (a–d) Tissue localization of DAO and 3MST. Western blot analysis was performed with antibodies against DAO (a,b) and 3MST (c,d) for the brain (a,c) and peripheral tissues (b,d). Relative amounts analysed by NIH Image J are shown in the upper column. **P<0.01. (e,f) H2S-producing activities fromD-cysteine andL-cysteine in the brain (e) and kidney (f). Homogenates were incubated with 10 mMD-cysteine orL-cysteine. **P<0.01. (g,h) The developmental changes in the levels of DAO and 3MST. Western blot analysis was performed and analysed by using NIH image J. (i,j) H2S production fromD-cysteine andL-cysteine. Homogenates were incubated with 10 mMD-cysteine orL-cysteine. (g–j) *P<0.05; **P<0.01; versus 0 week of each group. All data are expressed as the mean±s.e.m. of three experiments. Bs, brain stem; Ce, cerebrum; Cb, cerebellum; Di, diencephalon; He, heart; Ki, kidney; Li, liver; LI, large intestine; Lu, lung; Ov, ovary; Sp, spleen; SI, small intestine; Sm, skeletal muscle. Figure 2 Tissue localization of DAO and 3MST and developmental changes in H 2 S production. ( a – d ) Tissue localization of DAO and 3MST. Western blot analysis was performed with antibodies against DAO ( a , b ) and 3MST ( c , d ) for the brain ( a , c ) and peripheral tissues ( b , d ). Relative amounts analysed by NIH Image J are shown in the upper column. ** P <0.01. ( e , f ) H 2 S-producing activities from D- cysteine and L- cysteine in the brain ( e ) and kidney ( f ). Homogenates were incubated with 10 mM D- cysteine or L- cysteine. ** P <0.01. ( g , h ) The developmental changes in the levels of DAO and 3MST. Western blot analysis was performed and analysed by using NIH image J. ( i , j ) H 2 S production from D- cysteine and L- cysteine. Homogenates were incubated with 10 mM D- cysteine or L- cysteine. ( g – j ) * P <0.05; ** P <0.01; versus 0 week of each group. All data are expressed as the mean±s.e.m. of three experiments. Bs, brain stem; Ce, cerebrum; Cb, cerebellum; Di, diencephalon; He, heart; Ki, kidney; Li, liver; LI, large intestine; Lu, lung; Ov, ovary; Sp, spleen; SI, small intestine; Sm, skeletal muscle. Full size image The production of H 2 S by isolated mitochondria and peroxisomes from D -cysteine was examined. The isolated cerebellar mitocondria and peroxisomes produced H 2 S from D -cysteine. As mitochondria contain CAT, the isolated mitochondria produced H 2 S from L -cysteine along with α-KG ( Supplementary Fig. S2a,c ). H 2 S production from D -cysteine was greater than from L- cysteine along with α-KG in the presence of the isolated kidney mitochondria and peroxisomes ( Supplementary Fig. S2b,c ). H 2 S production from L -cysteine alone was undetectable in the presence of isolated mitochondrial and peroxisomes of both tissues. Developmental changes in H 2 S production We then examined the production of H 2 S from D- cysteine and L- cysteine and the expression of 3MST and DAO in the cerebellum and the kidney during development. In the cerebellum, the levels of DAO increased from birth until the mice were 8 weeks old, while the 3MST levels were relatively high at birth and only slightly decreased after 8 weeks ( Fig. 2g ). H 2 S production from D- cysteine increased over time, reaching the maximum production after 6 weeks, and then, it decreased, whereas H 2 S production from L- cysteine was much less and did not significantly vary over time ( Fig. 2i ). Similar results were obtained in the kidney ( Fig. 2h ). These observations suggest that the altered production of H 2 S from D- cysteine observed during development correlates well with the levels of DAO and 3MST, both in the cerebellum and the kidney. Increase in bound sulfane sulphur by D- cysteine administration Bound sulfane sulphur is the major physiologically relevant pool of H 2 S capable of regulating enzyme activity and cell growth [24] . As H 2 S produced from L- cysteine is stored as bound sulfane sulphur [14] , H 2 S produced from D- cysteine may also be stored. To examine this possibility, we orally administered D- cysteine to mice and measured the amount of bound sulfane sulphur in the cerebellum, cerebrum and kidney. The levels of bound sulfane sulphur in the cerebellum increased by 212% compared with the control 0.5 h after the administration of D- cysteine, and returned to the control level after 3 h; comparatively, L- cysteine did not significantly increase the levels of bound sulfane sulphur ( Fig. 3a ). Neither D- cysteine nor L- cysteine affected the cerebrum ( Fig. 3b ). D- Cysteine increased the levels of bound sulfane sulphur in the kidney by 236%, 218% and 196% at 0.5, 3 and 6 h after administration, respectively. L-C ysteine increased the levels by 172% after 0.5 h, but they immediately declined thereafter ( Fig. 3c ). These observations suggest that D- cysteine more efficiently increased the levels of bound sulfane sulphur than L- cysteine in the cerebellum and the kidney. 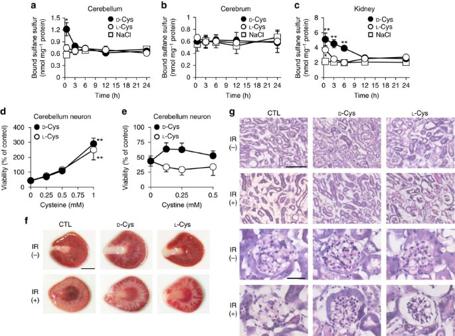Figure 3 D-Cysteine increases bound sulfane sulphur and protects cerebellar neurons and kidney. (a–c) Concentrations of bound sulfane sulphur after administration ofD-orL-cysteine. Tissues were obtained from mice at the times indicated after the administration ofD-orL-cysteine. *P<0.05; **P<0.01. (d,e) The protection of cerebellar neurons from H2O2-induced oxidative stress byD-orL-cysteine (d) andD-orL-cystine (e). The viability of cultured neurons was assessed by WST-8 assay. (f,g) Protection of the kidney from ischaemia-reperfusion injury byD-orL-cysteine. Kidney slices were stained with TTC (f, scale bar, 3 mm) or Periodic-Acid-Schiff (PAS) (g) 24 h after the ischaemia-reperfusion (IR) injury with or without the oral administration ofD-orL-cysteine. The structure of the renal cortex (g, upper two columns, scale bar, 400 μm) and that of glomerulus on a magnified scale (g, lower two columns, scale bar, 40 μm) were shown. All data are represented as the mean±s.e.m. of at least three experiments. Figure 3 D- Cysteine increases bound sulfane sulphur and protects cerebellar neurons and kidney. ( a – c ) Concentrations of bound sulfane sulphur after administration of D- or L- cysteine. Tissues were obtained from mice at the times indicated after the administration of D- or L- cysteine. * P <0.05; ** P <0.01. ( d , e ) The protection of cerebellar neurons from H 2 O 2 -induced oxidative stress by D- or L- cysteine ( d ) and D- or L- cystine ( e ). The viability of cultured neurons was assessed by WST-8 assay. ( f , g ) Protection of the kidney from ischaemia-reperfusion injury by D- or L- cysteine. Kidney slices were stained with TTC ( f , scale bar, 3 mm) or Periodic-Acid-Schiff (PAS) ( g ) 24 h after the ischaemia-reperfusion (IR) injury with or without the oral administration of D- or L- cysteine. The structure of the renal cortex ( g , upper two columns, scale bar, 400 μm) and that of glomerulus on a magnified scale ( g , lower two columns, scale bar, 40 μm) were shown. All data are represented as the mean±s.e.m. of at least three experiments. Full size image D- cysteine protects neurons from oxidative stress As H 2 S protects neurons from oxidative stress [8] , [9] , we examined whether D -cysteine protects cultures of cerebellar neurons from hydrogen peroxide (H 2 O 2 )-induced oxidative stress caused using 4-3-(2-methoxy-4-nitrophenyl)-2-(4-nitrophenyl)-2H-5-tetrazolio-1,3-benzene disulfonate sodium salt (WST-8) assay, a tetrazolium salt, which is reduced by cellular activity to form intensely coloured formazans, and have often used to quantitate the number of living cells. Fifty micromolar H 2 O 2 caused ~60% neuronal cell death 21 h after the application. The simultaneous application of D -cysteine with H 2 O 2 -protected neurons from H 2 O 2 -induced toxicity in a concentration-dependent manner ( Fig. 3d ). Both D - and L- cysteine at 1 mM increased the viability above 200% of a control. The oxidized form of D -cysteine, D -cystine, protected neurons greater than L- cystine, which is a major form in the extracellular fluid such as blood ( Fig. 3e ). D- cysteine protects the kidney from ischaemia-reperfusion injury We also examined the effect of D -cysteine on ischaemia-reperfusion injury in the kidney. The staining with 2, 3, 5-triphenyltetrazolium chloride (TTC), which is another tetrazolium salt, showed that the cortex was stained in mice orally administered D -cysteine, while it was not stained 24 h after ischaemia-reperfusion in control mice, suggesting that D -cysteine protects the renal cortex ( Fig. 3f ). TTC staining in the renal cortex in mice administered D- cysteine was greater than that in mice administered L -cysteine, suggesting that D- cysteine protects the renal cortex more efficiently than L -cysteine does. These observations were confirmed by Periodic-Acid-Schiff staining. The structure of the renal cortex was disintegrated after ischaemia-reperfusion ( Fig. 3g ). In contrast, it was well preserved in mice administered D -cysteine. The structure of glomeruli showed a significant difference from that of a control. In mice administered L -cysteine, glomeruli were shrunk and a wide space was observed between glomerulus and the surrounding capsule ( Fig. 3g ). These observations suggest that D -cysteine increases the levels of bound sulfane sulphur to protect the kidney from the ischaemia-reperfusion injury more efficiently than L -cysteine ( Fig. 3c ). Serum creatinine levels, which are increased by renal injury, were measured after the ischaemia-reperfusion of unilateral kidney. The ischaemia-reperfusion significantly increased serum creatinine, and D- cysteine decreased the level of serum creatinine more efficiently than L -cysteine but the difference was not statistically significant ( Supplementary Fig. S3 ). Sources of D- cysteine There are at least two possible sources of D- cysteine, namely, racemase-induced chiral change of L- cysteine and absorption from food. As cysteine is structurally similar to serine with an OH replaced by an SH, and because aspartate racemase is homologous to CAT, which has an affinity for both aspartate and cysteine [25] , [26] , [27] , it is possible that serine racemase or aspartate racemase changes L- cysteine to D- cysteine. However, we determined that neither recombinant racemase was capable of this conversion ( Supplementary Fig. S4 ). We also examined the racemase activity in the brain. The cerebellar homogenates produced a substance from L- cysteine detected at a retention time of 6.98 min after 30 min, and the peak was shifted to 6.93 min after 60-min incubation ( Supplementary Fig. S5b,c ). However, considering the difference in the retention time, we determined that neither peak was identical to D- cysteine (6.34 min), ( Supplementary Fig. S5e ). L- Amino acids are nonenzymatically racemized by heat and alkaline conditions applied during food processing, and 21–44% of L- cysteine is changed to D- cysteine by alkaline treatment [28] , [29] . D -cysteine may thus be mostly provided from food. Although D -cysteine was not detected in tissues after the oral administration, the levels of bound sulfane sulphur were increased to protect the kidney from ischaemia-reperfusion injury ( Fig. 3 ). These observations with the previous finding that D- cysteine is easily absorbed through the gastrointestinal tract and enters the blood stream [30] suggest that D- cysteine may be immediately metabolized to produce bound sulfane sulphur in tissues. Both D -cysteine and L -cysteine protect cerebellar neurons from oxidative stress, and further increase cell viability at the higher concentrations ( Fig. 3d ). Our previous study similarly showed that H 2 S specifically increased cell viability of neuronal cells [31] . D -Cystine protected cerebellar neurons more efficiently than L -cystine ( Fig. 3e ). It is probably because the transport activity for D -cystine is greater than that for L -cystine when compared at the same concentrations [32] . D -cysteine protects the renal cortex more efficiently than L -cysteine ( Fig. 3f ). As H 2 S-producing enzymes, CBS, CSE and 3MST along with DAO are localized to the renal cortex [33] , [34] , [35] , [36] , the administration of D -cysteine or L -cysteine protects the renal cortex but not the medulla ( Fig. 3f ). D -cysteine, which increases the levels of bound sulfane sulphur more greatly than L -cysteine, more efficiently protects the renal cortex than L -cysteine does ( Fig. 3f ). The observation also confirms the interaction between mitochondrial 3MST and peroxisomal DAO in vivo . L- Cysteine is an excitotoxin comparable in potency to other excitatory amino acids [37] . In contrast, the subcutaneous administration of D- cysteine does not cause excitotoxic damage to the brain [38] . Therefore, systemic application of D- cysteine may be less toxic than that of L- cysteine. The administration of D- cysteine may provide a new therapeutic approach to protect specific cells from oxidative stress or ischaemia-reperfusion injury through its conversion to H 2 S via a novel pathway with 3MST and DAO. Determination of H 2 S-producing activity All animal procedures were approved by the National Institute of Neuroscience Animal Care Use Committee. Whole-brain extracts were prepared from male C57BL/6N mice (Clea Japan, Tokyo, Japan) with nine volumes of ice-cold buffer A (100 mM potassium phosphate buffer (pH 7.4), 1 mM dithiothreitol (DTT), and a complete protease inhibitor cocktail (Roche Diagnostics, Mannheim, Germany)) by using a Potter-type glass homogenizer with a Teflon pestle or a Polytron-type homogenizer. To examine the stability of the enzymes following a single freeze-thaw cycle, the whole brain was immediately frozen at −80 °C after excision and thawed on ice. The extracts of the frozen-and-thawed tissue were prepared as described above. Enzymatic production of H 2 S was measured by following our previously described method [10] . Subcellular fractionation Whole-mouse brains were homogenized with three volumes of the fractionation buffer (5 mM MOPS (pH 7.4), 0.32 M sucrose, 1 mM EDTA, 0.1% ethanol and protease inhibitor cocktail) by using a Potter-type glass homogenizer with a Teflon pestle (1,200 r.p.m., three strokes) and centrifuged at 1,000 g for 10 min. The pellet was rehomogenized as described above and centrifuged twice at 600 g for 10 min. The final pellet was recovered as a nuclear fraction that was resuspended in fractionation buffer at 10% of the original volume. The post-nuclear supernatant was centrifuged at 16,500 g for 30 min to obtain the cytosolic and mitochondrial fractions. The mitochondrial pellets were resuspended in a volume of fractionation buffer equivalent to the supernatant. Determination of 3MP The mitochondrial pellets were resuspended in 10% of the original volume with 100 mM potassium phosphate buffer (pH 7.4) and a complete protease inhibitor cocktail. For the enzyme reactions, 11 μl of D- cysteine was added to 0.1 ml of the mitochondrial fraction to the final concentrations indicated in the figure legend and the reaction mixture was incubated at 37 °C for 50 min. The thiol group of 3MP is highly reactive and can form dimers in multiple combinations through interactions with itself and other thiols [39] . To block the reactivity, an equal volume of 0.1 M N -ethylmaleimide, which is a thiol-alkylating agent, was added to the mixture and incubated at 37 °C for 10 min. After centrifugation at 12,000 g for 10 min, the supernatant was centrifuged through Amicon Ultra centrifugal filters (Millipore, Bedford, MA) with a cutoff of 3 kDa. The alkylated 3MP in the filtrate was determined by the pre-labelling high-performance liquid chromatography assay using 1,2-diamino-4,5-dimethoxybenzene [40] . Western blot analysis The protein samples (10 μg) were fractionated by SDS–PAGE on a 12 or 15% polyacrylamide gel (DRC, Tokyo, Japan) and transferred to a polyvinylidene difluoride membrane (Millipore). The membrane was blocked by using PBS-T (137 mM NaCl, 10 mM Na 2 HPO 4 , 2.7 mM KCl, 1.8 mM KH 2 PO 4 and 0.1% Tween 20) containing 2% skim milk (Wako, Osaka, Japan) overnight at 4 °C and incubated with either anti-MPST (1:3,000; Atlas Antibodies AB, Stockholm, Sweden) or anti-DAO [41] (BioResource room, The Institute for Enzyme Research, The University of Tokushima) at 4 °C for 4 h. After additional 2-h incubation with the secondary anti-rabbit antibodies conjugated with horseradish peroxidase diluted at 1:20,000 (GE Healthcare), the binding of the antibodies was visualized using the Millipore Immobilon Western Chemiluminescent HRP substrate (Millipore) or Western Lightning ECL Pro (PerkinElmer, Waltham, MA). Cell culture Primary cerebellar neurons were prepared from embryonic day 16 imprinting control region (ICR) mice (Clea Japan). The cerebellum was digested with 0.25% trypsine and 0.1% DNase I in Ca 2+ /Mg 2+ -free PBS for 10 min at 37 °C. After pipetting cells were seeded on poly- D- lysine-coated 96-well microtiter dishes at 100,000 cells per 100 μl in each well. The cells were cultured in Neurobasal medium (Life technologies, Carlsbad, CA) supplemented with B27, 0.5 mM L- glutamine, 100 U ml −1 penicillin and 100 μg ml −1 streptomycin at 37 °C in 10% CO 2 . For the toxicity study, 5-day-old cells were exposed to 50 μM H 2 O 2 , and then cysteine or cystine was added to the concentrations indicated in the figure legend. WST-8 (2-(2-methoxy-4-nitrophenyl)-3-(4-nitrophenyl)-5-(2,4-disulfophenyl)-2H-tetrazolium, monosodium salt) viability assay was performed with the cell-counting kit-8 (Dojindo, Kumamoto, Japan) 21 h after the application of H 2 O 2 . Ten microliters of WST-8 was added to each well, cells were incubated at 37 °C for 2 h and absorption values at 450 nm were determined using a microplate reader. Values of samples were normalized by subtracting values of direct reduction of WST-8 by the chemicals. Administration of cysteine Male ICR mice (Clea Japan) with a body weight of 30–40 g were housed with ad libitum access to food and water. The animals were divided into three groups: D- cysteine, L- cysteine and control. The D- and L- cysteine (8 mmol kg −1 body weight) were orally administered by gastric intubation. The cysteine solution was adjusted to pH 2.0–2.5 with 5 M NaOH. The control mice received the same amount of NaCl. At the times indicated in the figure legend after oral administration, the mice were transcardially perfused with saline. The tissues were immediately removed, frozen with liquid nitrogen and then stored at −80 °C until the bound sulfane sulphur was measured. Determination of bound sulfane sulphur To determine the amount of bound sulfane sulphur, the frozen tissues were thawed on ice and homogenized with ice-cold lysis buffer B (10 mM potassium phosphate buffer (pH 7.4), 1% TritonX-100 and the protease inhibitor cocktail) with 10 mM of hydroxylamine and sodium benzoate (each), which suppress the activities of PLP-dependent enzymes and DAO that are involved in enzymatic H 2 S production. The lysates were centrifuged at 12,000 g for 10 min, and the supernatant was recovered. For measurement of the H 2 S released from the bound sulfane sulphur, 0.1 ml of sample (2.5 mg protein per ml) and 0.1 ml of 15 mM DTT in 0.2 M Tris/HCl (pH 9.0) were placed in a 15-ml centrifugation tube, sealed with Parafilm and then incubated at 37 °C for 50 min. After adding 0.4 ml of 1 M sodium citrate buffer (pH 6.0), the mixtures were incubated at 37 °C for 10 min with shaking at 125 rpm on a rotary shaker NR-3 (Taitec) to facilitate the release of H 2 S gas from the aqueous phase. H 2 S concentration was determined according to the method described for the determination of the H 2 S produced by the enzymes. A reaction mixture without the samples was used as a control to account for the release of H 2 S from DTT. Renal ischaemia-reperfusion Male ICR mice were anesthetized with an intraperitoneal injection of sodium pentobarbital (65 mg kg −1 body weight). Body temperature was maintained with a heating blanket. Male ICR mice with a body weight of 30–40 g were divided into three groups: D- cysteine, L- cysteine and a control. The D- and L- cysteine (8 mmol kg −1 body weight) were orally administered 30 min before ischaemia. Unilateral renal blood flow was interrupted for 30 min by clamping a nontraumatic vascular clamp over renal pedicles. The control mice were subjected to the same surgical procedures without the oral administration. Evaluation of ischaemia-reperfusion injury Twenty-four h after reperfusion, the kidney was sliced coronally into 2-mm-thick sections by a tissue slicer. To visualize the area of the ischaemia-reperfusion injury, the slices were incubated with 2% TTC in saline at room temperature for 30 min. For histological analysis with a light-microscopy, mice were perfused with 4% (w/v) paraformaldehyde transcardially. The kidney was removed, post-fixed in paraformaldehyde at 4 °C overnight and immersed in 5, 15 and 30% (w/v) sucrose in order at 4 °C. The kidney was then submerged into an O.C.T. compound and frozen. The kidney sections with 4 μm thickness were cut by a cryostat at −20 °C. The sections were stained with Periodic-Acid-Schiff to highlight glomerular capillary loops and tubular epithelium. Stained sections were observed with an Axiophoto microscope (Carl Zeiss, Jena, Germany) equipped with a cooled CCD digital camera (Penguin 600CL; Pixera, Los Gatos, CA). Statistics All statistical analyses of the data were performed using Excel 2007 with the add-in software Statcel2 (OMS, Saitama, Japan). Differences between three or more groups were analysed with one-way analysis of variance. Post hoc multiple comparisons were made using the Bonferroni test. How to cite this article: Shibuya, N. et al. A novel pathway for the production of hydrogen sulfide from D- cysteine in mammalian cells. Nat. Commun. 4:1366 doi: 10.1038/ncomms2371 (2013).